Pollen tube emergence is mediated by ovary-expressed ALCATRAZ in cucumber 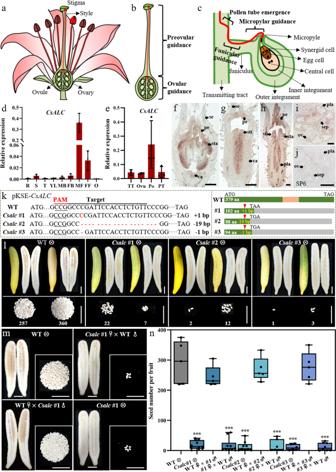Fig. 1:CsALCexpression pattern in reproductive organs and defective female fertility ofCsalcmutants by CRISPR-Cas9. a–cSchematic diagram of pollen tube guidance during the process of fertilization in flowering plants.aSchematic diagram of a flower showing the pollen tube penetrates through the stigma and style, enters the ovary, and targets an ovule.bTwo phases of pollen tube guidance: preovular guidance and ovular guidance.cOne pollen tube emerges from the transmitting tract (pollen tube emergence process) by ovule attraction, then extends towards the embryo sac under funicular guidance and micropylar guidance.d,eqPCR analysis ofCsALCexpression in different cucumber organs. R roots, S stems, T tendrils, YL young leaves, MB male flower buds, FB female flower buds, MF male flowers, FF female flowers, O ovaries at anthesis, TT ovary transmitting tract at anthesis, Ovu ovules at anthesis, Po pollens at anthesis, PT pollen tubes at 3 h after germination. The vertical axis refers to the relativeCsUBI(CsaV3_5G031430) expression.n= 3 biologically independent samples. Error bars represent mean ± SD.f–jIn situ hybridization ofCsALCin cucumber flower buds.fA male flower bud at stage 9.g,hLongitudinal sections of female flower buds at stage 8-1 (g), and 8-2 (h).iOvary transection of a female flower bud at stage 9.jOvary transection of a female flower bud at stage 8 hybridized with sense probe ofCsALCas the negative control. se sepal, pe petal, sta stamen, sti stigma, ca carpel, pla placenta, sep septum, ov ovule. Scale bars = 200 μm. The experiment was repeated three times with similar results.kMutation forms of three homozygous T1Csalcmutant lines by CRISPR-Cas9 system. The target sequence and PAM are marked by a black line and a red line, respectively. Deletions/ insertions are indicated as red dashes/ nucleotides, and corresponding nucleotide sizes are marked after the sequence as a minus or plus, respectively. The right dotted box shows the corresponding protein premature termination. The green/gray boxes indicate the protein-coding region and missense sequences resulting from frameshift mutations, respectively. The orange box in WT represents the bHLH conserved domain in CsALC. aa amino acid.lSeed number of wild type (WT) andCsalcmutant lines by self-pollination. Pictures represent the mature fruit, its longisection, and all plump seeds harvested from it, with the corresponding number at the bottom. Scale bars = 5 cm.mReciprocal cross betweenCsalc#1 mutant and WT. Scale bars = 5 cm. The experiments were repeated three times with similar results (l,m).nQuantitative analysis of seed numbers from (l,m). Upmost/lowest lines indicate the maximum/minimum values, box limits indicate the upper and lower quartiles, and lines in boxes indicate the median values of these data. From left to right,n= 5, 11, 5, 10, 9, 5, 7, 6, 5, 8 mature fruits. ***p< 0.001, compared to WT (two-sided Student’st-test). Pollen tube guidance within female tissues of flowering plants can be divided into preovular guidance, ovular guidance and a connecting stage called pollen tube emergence. As yet, no female factor has been identified to positively regulate this transition process. In this study, we show that an ovary-expressed bHLH transcription factor Cucumis sativus ALCATRAZ (CsALC) functions in pollen tube emergence in cucumber. CsALC knockout mutants showed diminished pollen tube emergence, extremely reduced entry into ovules, and a 95% reduction in female fertility. Further examination showed two rapid alkalinization factors CsRALF4 and CsRALF19 were less expressed in Csalc ovaries compared to WT. Besides the loss of male fertility derived from precocious pollen tube rupture as in Arabidopsis , Csralf4 Csralf19 double mutants exhibited a 60% decrease in female fertility due to reduced pollen tube distribution and decreased ovule targeting efficiency. In brief, CsALC regulates female fertility and promotes CsRALF4/19 expression in the ovary during pollen tube guidance in cucumber. Seed production is critically important for sexual propagation in agricultural crops. Successful delivery of sperm cells (contained within the pollen tube) to female gametes enclosed inside the ovary is a prerequisite for seed genesis [1] , [2] , [3] . After germinating on the stigma, pollen tubes extend and navigate along the female reproductive tract (transmitting tract: TT) towards ovules [1] , [4] (Fig. 1a ). During this process, the pollen tube perceives signal substances from both female sporophytic and gametophytic tissues of the pistil, which guide it towards the embryo sac, where the pollen tube penetrates into the synergid and releases two sperm cells, with one fusing with the egg cell and the other with the central cell [5] , [6] . Pollen tube guidance can be divided into preovular guidance (before entering into the ovary) and ovular guidance (Fig. 1b ); the latter step is further divided into funicular guidance (guidance from the septum surface to the funiculus) and micropylar guidance (guidance from funiculus to micropyle and embryo sac) (Fig. 1c ) [5] , [7] , [8] . Between preovular and ovular guidance, there is a crucial transition phase called pollen tube emergence, in which pollen tubes exit from the transmitting tract and move onto the septum surface (Fig. 1c ). Fig. 1: CsALC expression pattern in reproductive organs and defective female fertility of Csalc mutants by CRISPR-Cas9. a–c Schematic diagram of pollen tube guidance during the process of fertilization in flowering plants. a Schematic diagram of a flower showing the pollen tube penetrates through the stigma and style, enters the ovary, and targets an ovule. b Two phases of pollen tube guidance: preovular guidance and ovular guidance. c One pollen tube emerges from the transmitting tract (pollen tube emergence process) by ovule attraction, then extends towards the embryo sac under funicular guidance and micropylar guidance. d , e qPCR analysis of CsALC expression in different cucumber organs. R roots, S stems, T tendrils, YL young leaves, MB male flower buds, FB female flower buds, MF male flowers, FF female flowers, O ovaries at anthesis, TT ovary transmitting tract at anthesis, Ovu ovules at anthesis, Po pollens at anthesis, PT pollen tubes at 3 h after germination. The vertical axis refers to the relative CsUBI (CsaV3_5G031430) expression. n = 3 biologically independent samples. Error bars represent mean ± SD. f – j In situ hybridization of CsALC in cucumber flower buds. f A male flower bud at stage 9. g , h Longitudinal sections of female flower buds at stage 8-1 ( g ), and 8-2 ( h ). i Ovary transection of a female flower bud at stage 9. j Ovary transection of a female flower bud at stage 8 hybridized with sense probe of CsALC as the negative control. se sepal, pe petal, sta stamen, sti stigma, ca carpel, pla placenta, sep septum, ov ovule. Scale bars = 200 μm. The experiment was repeated three times with similar results. k Mutation forms of three homozygous T1 Csalc mutant lines by CRISPR-Cas9 system. The target sequence and PAM are marked by a black line and a red line, respectively. Deletions/ insertions are indicated as red dashes/ nucleotides, and corresponding nucleotide sizes are marked after the sequence as a minus or plus, respectively. The right dotted box shows the corresponding protein premature termination. The green/gray boxes indicate the protein-coding region and missense sequences resulting from frameshift mutations, respectively. The orange box in WT represents the bHLH conserved domain in CsALC. aa amino acid. l Seed number of wild type (WT) and Csalc mutant lines by self-pollination. Pictures represent the mature fruit, its longisection, and all plump seeds harvested from it, with the corresponding number at the bottom. Scale bars = 5 cm. m Reciprocal cross between Csalc #1 mutant and WT. Scale bars = 5 cm. The experiments were repeated three times with similar results ( l , m ). n Quantitative analysis of seed numbers from ( l , m ). Upmost/lowest lines indicate the maximum/minimum values, box limits indicate the upper and lower quartiles, and lines in boxes indicate the median values of these data. From left to right, n = 5, 11, 5, 10, 9, 5, 7, 6, 5, 8 mature fruits. *** p < 0.001, compared to WT (two-sided Student’s t -test). Full size image Accurate pollen–pistil interactions occur during the long journey from stigma to ovules, functional disruption of either male gametophytes or female reproductive tissues will bring obstacles to oriented pollen tube growth, and thus lead to failure of double fertilization [9] . Upon landing on the stigma, Arabidopsis compatible pollen grains germinate via precise interactions between the pollen and pistil involving POLLEN COAT PROTEIN B-class peptides and ANJEA-FERONIA receptor kinase complex [10] . In tomato ( Lycopersicon esculentum ), LeSTIG1, a cysteine-rich protein secreted from the pistil, can bind to the pollen-specific receptor kinases LePRK1 and LePRK2 to stimulate pollen tube growth [11] . Arabidopsis pollen tube-specific cysteine-rich peptides (CRPs), Rapid Alkalinization Factor 4 (RALF4), and RALF19 [12] , [13] , together with their pollen tube located Catharanthus roseus Receptor Like Kinase 1 Like (CrRLK1L) receptors BUDDA’S PAPER SEAL1 (BUPS1)/ BUPS2 [12] , and ANXUR1 (ANX1)/ ANX2 [14] , [15] , and co-receptors glycosylphosphatidylinositol-anchored proteins (GPI-APs), LORELEI-like-GPI-anchored protein 2 (LLG2) and LLG3 [16] , are demonstrated to control pollen tube integrity and growth. Pollen tubes in double mutant ralf4 ralf19 [12] , [13] , anx1 anx2 [14] , [15] , bups1 bups2 [12] , llg2 llg3 [16] all burst precociously at stigma or not beyond the style, resulting in extension cutoff at preovular stage. “Ovular guidance” attracts one pollen tube to its target ovule, forming a specific one-to-one relationship [5] . Besides Arabidopsis MAGATAMA1 (MAA1: an unknown type protein) and MAA3 (a kind of helicase) [8] , [17] , several attractant peptides produced from female gametophytes have been identified to govern ovular guidance, including the Gramineae-specific small peptide EGG APPARATUS1 (EA1) in maize [18] , [19] , defensin-like CRPs LUREs and XIUQIUs in Torenia fournieri [20] and Arabidopsis [21] , [22] . In Arabidopsis , the leucine-rich repeat receptor-like kinase (LRR-RLK) PRK6, localized at the pollen tip, was identified as the receptor for LURE1s [23] . Unlike that knock-down of EA1 gene resulted in ovule sterility in maize, neither Arabidopsis allure1 septuple mutants nor prk6 mutant exhibited defects in fertility. Simultaneous knockout of both 7 LURE1s and 4 XIUQIUs led to only a 20% decrease in female fertility, indicating the redundant roles between LURE1s and XIUQIUs, and additional attractants in Arabidopsis micropylar guidance [22] , [24] . Pollen tube emergence as the transition phase between preovular and ovular guidance refers to the first re-orientation of pollen tubes extending from the transmitting tract to the septum surface before proceeding onto funiculus, which was speculated to be affected by ovules to some extent [5] . In Arabidopsis, pollen tubes that lost the function of two endoplasmic reticulum-localized cation/proton exchangers CHX21 and CHX23 exhibited normal growth but were unable to emerge from the transmitting tract, showing a defect in pollen tube guidance [25] . Recently, pollen tube-expressed RALF6, 7, 16, 36, and 37 were shown to interact with female tissue-located receptor-like kinases FERONIA, ANJEA, and HERCULES RECEPTOR KINASE 1 (HERK1) to control the emergence of a single pollen tube at the septum for each ovule [26] . The multiple mutants of RALFs or RLK genes showed polytubey phenotype (arrival of multiple pollen tubes to one ovule) [26] . Although it was proposed there exists long-range attraction from ovules, no female sporophytic genes have been identified to positively regulate pollen tube emergence in planta so far [5] . ALCATRAZ ( ALC ) encodes a bHLH transcription factor that mediates fruit opening by driving the formation of a separation layer at the valve/replum border that constitutes the dehiscence zone with the lignified layer in Arabidopsis [27] . Cucumber ( Cucumis sativus L.) is an important vegetable crop bearing pepo fruit cultivated worldwide for over 3000 years [28] . In this study, we found cucumber ALC homolog (CsALC) functioned specifically in pollen tube emergence, regulated female fertility, and promoted TT-expressed CsRALF4/19 during pollen tube growth in cucumber. CsALC is highly expressed in reproductive organs of cucumber To identify putative fruit developmental regulators in the fleshy pepo fruit, the cucumber homolog of Arabidopsis bHLH transcription factor ALC, functioning in fruit opening, was searched in Cucurbit Genomics Database (CuGenDB: http://cucurbitgenomics.org/ ), and named as CsALC (Csa2G356640.1). ALC was reported to be the closest relative to SPATULA (SPT) [29] . Phylogenetic analysis showed there were SPT lineage and ALC lineage within core eudicots (Supplementary Fig. 1a ). CsALC gene contains six exons and five introns, and its encoded protein is located in the nucleus, with 379 amino acids and a typical bHLH domain (Supplementary Fig. 1b–d ). qPCR analysis showed that CsALC transcripts accumulate predominately in reproductive organs, including male flowers and female flowers (Fig. 1d ). During fertilization, CsALC was expressed in transmitting tract (TT), ovules, pollens, and pollen tubes (Fig. 1e ). In situ hybridization further localized CsALC transcripts in petals, stamens, and degenerated carpel primordia in male flower buds (Fig. 1f ). In female flower buds, there was substantial enrichment of CsALC signals in developing carpels, especially placenta and stigmas, as well as in petals and degraded stamen primordia (Fig. 1g, h ). Ovary transverse sections showed that compared to the negative control, prominent CsALC signals were localized in ovules, placenta, and septum (two parts where transmitting tracts are generated for fertilization in cucumber) at female flower bud stage (Fig. 1i, j ). Knockout of CsALC resulted in reduced female fertility in cucumber To gain insight into CsALC function in cucumber, the first exon of CsALC was targeted by CRISPR-Cas9 gene-editing system (Supplementary Fig. 1b ). Three homozygous frameshift mutant lines were obtained for further characterization (Fig. 1k ). Compared to the wild type (WT), Csalc mutant lines exhibited similar plant growth and fruit length (Supplementary Fig. 2a–c ). 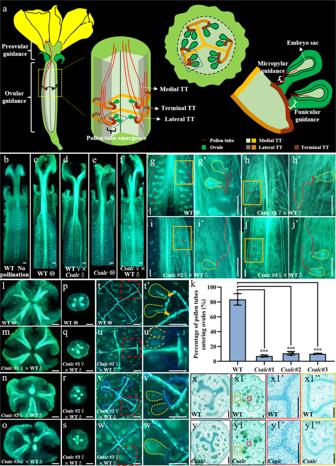Fig. 2: Pollen tubes are less likely to reach ovules in theCsalcovary. aSchematic diagram of pollen tube paths along the female reproductive tract in cucumber, in which the ovary transmitting tract (TT) consists of medial TT [pale green (longitudinal section) and orange (transverse section)], lateral TT [gray (longitudinal section) and light brown (transverse section)] and terminal TT (dark brown).b–fLongitudinal sections showing pollen tubes extend along the transmitting tract from top to bottom in WT andCsalcovaries. Composite images were integrated and spliced from local images taken separately. Scale bars = 500 μm.g–j’Typical images showing WT pollen tubes enter ovules in WT andCsalcmutants by longitudinal sections. Red arrow heads indicate pollen tubes targeting ovules.g’–j’Enlarged view of the orange boxes in (g–j). Targeted ovules are delineated by yellow dots, and pollen tubes are marked by red lines. Scale bars = 500 μm.kQuantitative analysis of pollen tubes entering ovules in WT andCsalcmutants.n= 3 biologically independent samples. Error bars represent mean ± SD. ***p< 0.001, compared to WT (two-sided Student’sttest).l–w’Transverse sections displaying the diminished distribution of pollen tubes at terminal transmitting tract inCsalcovaries, and pollen tubes unable to target ovules.l–ostigma,p–sstyle,t–wthe top quarter of the ovary.t’–w’Enlarged view of red dotted boxes in (t–w). The ovules are delineated by yellow dots. Orange arrows refer to pollen tubes entering ovules. Scale bars = 500 μm.x–y1”Cell morphology and structural composition of the transmitting tract in styles (x,y) and ovaries (x1,y1) of WT (top row) andCsalcmutant (bottom row) by Alcian blue staining. (x1’,y1’) and (x1”,y1”) are enlargement of red and orange boxes in (x1) and (y1), respectively. Scale bars = 200 μm. However, the seed number per fruit in Csalc mutant lines was dramatically reduced after self-pollination (Fig. 1l ), and the few seeds were randomly distributed in the fruit chamber of Csalc mutants. Considering the higher expression of CsALC in male gametophytes (Fig. 1e ), we first investigated the pollen development and viability by Alexander staining and in vitro germination assays. As shown in Supplementary Fig. 2d , Csalc pollen grains were morphologically normal and able to germinate and grow on a medium. Quantitative analysis showed the slightly reduced viability of Csalc pollens (90.4 ± 1.6%, 90.6 ± 1.7%, 90.6 ± 1.1%, p < 0.001 versus WT 97.9 ± 1.4% by Alexander staining assay; 94.9 ± 1.3% p < 0.01, 94.9 ± 0.7% p < 0.001, 95.2 ± 1.8% p < 0.05 versus WT 99.2 ± 0.5% by in vitro germination assay) (Supplementary Fig. 2e, f ). This mild decrease in pollen viability has a negligible impact on the cucumber seed set since an excess of pollens is usually available during open pollination. Next, reciprocal crosses between Csalc mutants and WT were performed. As shown in Fig. 1m, n , when Csalc pollens were pollinated to WT, high seed set was acquired (244.6 ± 35.3, 269.6 ± 39.5, 277.0 ± 49.6 seeds per fruit), similar to that in WT self-crossing (292.5 ± 70.9). In contrast, when Csalc mutants were fertilized with WT pollens, a drastically lower seed set (17.2 ± 22.1, 15.3 ± 19.2, 12.5 ± 13.3, p < 0.001 versus WT self-crossing) was obtained, equivalent to those in Csalc mutant self-pollination (18.3 ± 13.9, 13.7 ± 15.9, 11.0 ± 9.6, p < 0.001 versus WT self-crossing), resulting in an average of 95% (respective 94.1%, 94.8%, 95.7%) decrease in seed number per fruit compared to WT. The above data suggested Csalc mutants have a remarkable defect in female fertility. When a heterozygous+/ Csalc mutant self-crossing, the +/+, +/ Csalc , Csalc/Csalc in the 213 progeny seedlings showed segregation of 53:117:43, approximating the ratio of 1:2:1, suggesting that the defect in Csalc mutant is localized to female sporophytic tissues. Pollen tubes displayed difficulty in targeting ovules in Csalc mutants Successful fertilization in flowering plants requires accurate pollen tube guidance in pistils, which can be divided into preovular guidance, ovular guidance, and a transition phase called pollen tube emergence [5] . As shown in Fig. 2a , we illustrated these processes in cucumber. Unlike the dehiscent silique with two cavities in Arabidopsis , cucumber produces fleshy fruit, which is generally developed from three dorsally fused carpels, and the ovules encased by flesh are born at both edges of each carpel. The distinct carpel fusion form in cucumber gives rise to the unique morphology of the transmitting tract (TT), which is divided into medial TT, lateral TT, and terminal TT in ovary [30] (Fig. 2a ). After entering into ovaries, pollen tube bundles firstly extend along medial TT to the nearby lateral TT, then after a short extension, pollen tubes exit from lateral TT to terminal TT, resembling Arabidopsis pollen tube emergence process in which pollen tubes start to depart from the main growth axis to target ovules (Fig. 2a ). Therefore, this first re-orientation in cucumber is designated as “pollen tube emergence”. The second re-orientation from terminal TT to funiculus is depicted as funicular guidance (Fig. 2a ). After extremely short navigation along the funiculus, a third re-orientation is likely triggered by micropylar guidance cues at a much closer range from micropyle (Fig. 2a ). Fig. 2: Pollen tubes are less likely to reach ovules in the Csalc ovary. a Schematic diagram of pollen tube paths along the female reproductive tract in cucumber, in which the ovary transmitting tract (TT) consists of medial TT [pale green (longitudinal section) and orange (transverse section)], lateral TT [gray (longitudinal section) and light brown (transverse section)] and terminal TT (dark brown). b – f Longitudinal sections showing pollen tubes extend along the transmitting tract from top to bottom in WT and Csalc ovaries. Composite images were integrated and spliced from local images taken separately. Scale bars = 500 μm. g – j’ Typical images showing WT pollen tubes enter ovules in WT and Csalc mutants by longitudinal sections. Red arrow heads indicate pollen tubes targeting ovules. g’ – j’ Enlarged view of the orange boxes in ( g – j ). Targeted ovules are delineated by yellow dots, and pollen tubes are marked by red lines. Scale bars = 500 μm. k Quantitative analysis of pollen tubes entering ovules in WT and Csalc mutants. n = 3 biologically independent samples. Error bars represent mean ± SD. *** p < 0.001, compared to WT (two-sided Student’s t test). l – w’ Transverse sections displaying the diminished distribution of pollen tubes at terminal transmitting tract in Csalc ovaries, and pollen tubes unable to target ovules. l – o stigma, p – s style, t – w the top quarter of the ovary. t’ – w’ Enlarged view of red dotted boxes in ( t – w ). The ovules are delineated by yellow dots. Orange arrows refer to pollen tubes entering ovules. Scale bars = 500 μm. x – y1” Cell morphology and structural composition of the transmitting tract in styles ( x , y ) and ovaries ( x1 , y1 ) of WT (top row) and Csalc mutant (bottom row) by Alcian blue staining. ( x1’ , y1’ ) and ( x1” , y1” ) are enlargement of red and orange boxes in ( x1 ) and ( y1 ), respectively. Scale bars = 200 μm. Full size image To dissect the defective step of fertilization in Csalc mutants, Aniline blue staining was used to visualize pollen tube elongation and penetration in pistils. Compared to the WT ovary without pollination (Fig. 2b ), obvious fluorescence signals showed the movement trail of pollen tubes from the stigma to style, ovary chamber, and finally the ovules in WT self-crossing or hybridized with Csalc pollens (Fig. 2c, d ). In Csalc ovaries, pollen tubes spread normally downward along the medial transmitting tract and maintained similar fluorescence intensity with those in WT (Fig. 2e, f ). By local longitudinal sections, abundant pollen tubes could be observed emerging from lateral TT and entering ovules in WT (Fig. 2g–g ’), while rare in Csalc mutants (Fig. 2h–j ’). Quantitative analysis showed that 83.5 ± 7.7% pollen tubes successfully targeted ovules in WT, while only 7.1 ± 1.4%, 10.8 ± 2.4%, 10.1 ± 0.7% in Csalc #1, #2, #3 mutants, respectively (Fig. 2k ). Transverse sections of stigmas and styles showed comparable fluorescence intensity of pollen tubes at the stigma and style transmitting tract in Csalc mutants to that in WT (Fig. 2l–s ). While, the fluorescence signals in Csalc mutants were almost abolished at the terminal TT where funiculus attached (Fig. 2t–w ), and pollen tubes were barely observed approaching and penetrating into ovules as compared to WT (Fig. 2t’–w' ). By a time-course observation (2, 5, 10, 20 h), we found WT pollen tubes grew in Csalc transmitting tract at a similar rate to those in WT (Supplementary Fig. 3a ). However, pollen tubes at lateral TT extended almost downward, and rarely spread to terminal TT or turned growth direction to where ovules located in Csalc mutants (Supplementary Fig. 3b, c ). Therefore, the decreased female fertility in Csalc mutants is from the defect in pollen tube emergence from lateral TT to terminal TT. No difference was observed in tissue structure and cell morphology between Csalc mutant and WT transmitting tract, while the extracellular matrix (ECM) content in ovary TT detected by Alcian blue staining, an indicator of acidic polysaccharides, displayed a reduction in Csalc mutants (Fig. 2x–y1” ). ECM, containing various glycoproteins, has been proposed to mediate the attraction, nutrition, and stimulation of pollen tube growth in Arabidopsis [4] . CsRALF4/19 transcripts declined at the transmitting tracts in Csalc mutants To explore putative downstream targets of CsALC during fertilization, transcriptomic analyses were performed on WT and Csalc ovaries at 32 h after pollination (Supplementary Fig. 4a ). Differentially expressed genes (DEGs) were identified using the false discovery rate <0.05 and fold change larger than 2 as thresholds. A total of 8 and 20 genes were up- and down-regulated in Csalc ovaries, respectively (Supplementary Fig. 4b, c ). Among them, a gene encoding rapid alkalinization factor (Csa6G484570, CsRALF19 ) was remarkably decreased (log2 fold change = 3.46, P = 3.49E−04) in Csalc mutants (Supplementary Fig. 4d ). qPCR analysis using unpollinated ovary at anthesis showed that CsRALF19 and its paralogous gene CsRALF4 (Csa6G199790) were expressed significantly lower in Csalc mutants than WT (Fig. 3a, b ). Phylogenetic analysis indicated that the two peptides clustered with Arabidopsis RALF4/19, which function in pollen tube integrity (Supplementary Fig. 5a ) [12] , [13] . Unlike the pollen-specific expression of Arabidopsis RALF4/19 , CsRALF4/19 also have a certain degree of expression in the ovary, indicating their putative new function in female tissues in cucumber. CsRALF4 and CsRALF19 both contain a single exon and encode a 116- and a 112-amino-acid-long peptide, respectively (Supplementary Fig. 5b ). Fig. 3: Reduced transcript accumulation of CsRALF4 and CsRALF19 in Csalc ovaries. a , b Expression of CsRALF4 ( a ) and CsRALF19 ( b ) in unpollinated ovaries at anthesis of WT and Csalc mutants by qPCR. * p < 0.05, ** p < 0.01 (two-sided Student’s t -test). c , d CsRALF4 ( c ) and CsRALF19 ( d ) expression in different cucumber organs. S stems, MB male flower buds at stage 10 50 ; FB female flower buds at stage 10 50 ; O ovaries at anthesis; Sta stamens at anthesis. e , f CsRALF4 ( e ) and CsRALF19 ( f ) expression in female sporophytes and male gametophytes. TT ovary transmitting tract at anthesis, Ovu ovules at anthesis, Po pollens at anthesis, PT pollen tubes at 3 h after germination. The left/right vertical axis refers to the data of the blue/orange column, respectively, due to the magnitude difference of expression in different tissues. n = 3 biologically independent samples ( a–f ). The values were normalized with the CsUBI (CsaV3_5G031430) expression ( a-f ). Error bars represent mean ± SD ( a–f ). g–o’ Transcript accumulation of CsALC ( g , g’ , m , m’ ), CsRALF4 ( h , h’ , k , k’ , n , n’ ), and CsRALF19 ( i , i’ , l , l’ , o , o’ ) at transmitting tract of unpollinated WT and Csalc ovaries ( g–l’ ) and fertilized WT ovaries one day after anthesis (32 h after pollination) ( m–o’ ) by in situ hybridization. j – j’ SP6, Sense CsALC probe was hybridized as the negative control. g’–o’ are enlargements of red boxes in ( g–o ). Red arrows indicate transcript signals at lateral- and terminal-TTs in WT before pollination, and blue arrows refer to the weakened transcript signals at lateral- and terminal-TTs in Csalc mutants, or in WT after fertilization. Scale bars = 500 μm. The experiment was repeated three times with similar results. Full size image qPCR analysis showed that CsRALF4 / 19 were highly expressed in mature stamens (Fig. 3c, d ). However, unlike the differential expression of CsRALF4 / 19 in female tissues of Csalc mutants and WT, the expression of these two genes in stamens was unchanged between Csalc mutants and WT (Supplementary Fig. 6a, b ). Tissue subdivision showed that CsRALF4/19 transcripts were enriched in pollen grains and pollen tubes. Notably, the expression of CsRALF4/19 in the transmitting tract was higher than that in ovules (Fig. 3e, f ). To compare the expression pattern in WT and Csalc mutants, in situ hybridization of CsRALF4 / 19 and CsALC was performed on the transections of ovaries before pollination and after fertilization. In WT unpollinated ovaries, CsRALF4 / 19 and CsALC transcripts were enriched at transmitting tract and ovules (Fig. 3g–i’ ), and CsRALF19 exhibited much higher expression than CsRALF4 , consistent with qPCR results (Fig. 3e, f ). In Csalc unpollinated ovaries, CsRALF4/19 transcript signals seemed weaker at TTs compared to WT (Fig. 3k, l’ ). The TT identity and morphology appeared unaltered, and the TT marker gene SPATULA ( CsSPT ) was expressed normally in Csalc ovaries compared to WT [30] (Supplementary Fig. 6c ). Considering the almost abolished pollen tube extension to terminal TT in Csalc ovaries (Fig. 2g–w ), we speculated CsALC may regulate pollen tube emergence at least partially through CsRALF4/19 function in cucumber. While after fertilization, transcripts of all three genes showed reduced accumulation (Fig. 3m–o ’), indicating the potential specific roles of these genes in ovary TTs during the fertilization process. Positive regulation of CsALC on CsRALF4/19 expression To examine any direct regulation of CsALC on CsRALF4/19 expression, the cis-elements in CsRALF4/19 genes were analyzed. The bHLH transcription factor was shown to bind to the G-box of target genes [31] . G-box elements in the promoter of 28 DEGs between Csalc mutants and WT were searched on the PlantCARE website ( http://bioinformatics.psb.ugent.be/webtools/plantcare/html/ ) (Supplementary Data 4 ). CsRALF4 has one G-boxes in the promoter region, and one in the genomic region, and CsRALF19 has two G-box in the promoter region, and one in the genomic region (Supplementary Fig. 7a ). Yeast one hybrid (Y1H) assay showed that CsALC was unable to bind to any G-box containing fragments in CsRALF4 and CsRALF19 (Supplementary Fig. 7b ). However, using the complete promoter sequence (1811 bp for CsRALF4 and 3326 bp for CsRALF19 ), both pCsRALF4:LUC and pCsRALF19:LUC could be activated upon co-infiltration of CsALC protein in Nicotiana benthamiana leaves, increasing to 2.03 and 1.66 fold, respectively (Supplementary Fig. 7c ). These results indicated the positive regulation of CsALC on CsRALF4 / 19 expression in cucumber, consistent with the downregulation of CsRALF4 / 19 transcripts in Csalc mutants as detected by qRT-PCR and in situ hybridization (Fig. 3 ). Knockout of both CsRALF4 and CsRALF19 led to reduced female fertility and a complete loss of male fertility To characterize the function of CsRALF4/19 in cucumber, single mutants Csralf4 (obtained by targeting the CsRALF4 gene) and Csralf19 (separated from Csralf4 Csralf19 double mutants), as well as double mutant Csralf4 Csralf19 (generated by simultaneously targeting CsRALF4 and CsRALF19 ), were obtained by CRISPR-Cas9 system. Two homozygous lines for each mutant type were chosen for further characterization. Sequencing data showed that all mutant lines possessed frameshift mutations that resulted in protein premature termination (Figs. 4a, d, and 5a ). Both Csralf4 and Csralf19 single mutants showed a reduced seed set when self-crossing (seed number per fruit: Csralf4 mutants 219.6 ± 49.6, 203.0 ± 42.0, p < 0.05 versus WT 338.2 ± 101.6; Csralf19 mutants 217.0 ± 37.7, 227.7 ± 43.9, p < 0.05 versus WT 295.4 ± 61.7). When Csralf4 or Csralf19 mutant ovaries pollinated by WT pollens, seed numbers ( Csralf4 mutants as maternal parents: 337.9 ± 78.4 and 296.9 ± 49.0; Csralf19 mutants as maternal parents: 317.9 ± 81.6 and 300.0 ± 62.3) were comparable to WT self-crossing, suggesting the female fertility in both single mutants is normal. However, when Csralf4/ Csralf19 mutants as pollen donors to WT ovaries, the resultant seed set was significantly reduced (194.5 ± 62.8, 183.2 ± 38.5, p < 0.05 for Csralf4 mutants, and 214.4 ± 30.1, 226.5 ± 31.1, p < 0.05 for Csralf19 mutants) versus WT self-crossing, suggesting the defective male fertility in Csralf4 and Csralf19 single mutants (Fig. 4b, c, e, f ). Further, Csralf4 Csralf19 double mutants completely lost male fertility and none seed was produced when as pollen donors (Fig. 5b ). Intriguingly, when Csralf4 Csralf19 double mutants hybridized with WT pollens, the seed number per fruit (125 ± 51.3, 122.3 ± 63.8, p < 0.001) was significantly fewer than WT self-pollination (295.4 ± 61.7), accounting for ~60% decrease in female fertility (Fig. 5c, d ). The distribution of full seeds in the ovary chamber of Csralf4 Csralf19 double mutants was scattered, similar to that in Csalc mutants. The average seed number per unit fruit length (1 cm) in Csralf4 Csralf19 double mutants was 12.7 ± 4.5 ( p < 0.001) and 15.5 ± 7.1 ( p < 0.001), significantly reduced as compared to WT (29.6 ± 7.0) (Fig. 5c, e ). Moreover, only 38.5 ± 5.9% ( p < 0.001) and 37.7 ± 5.4% ( p < 0.001) ovules were observed to be targeted by pollen tubes in two Csralf4 Csralf19 double mutant lines, while the targeting ratio was 76.7 ± 8.1% in WT (Fig. 5f, g ). The pollen tube density at the lateral- and terminal-transmitting tract in Csralf4 Csralf19 ovaries was significantly reduced versus WT (Fig. 5h–j ). These data suggested a new role of CsRALF4 / 19 in female fertility in cucumber. Fig. 4: Decreased seed set in Csralf4 and Csralf19 single mutants. a , d Mutation forms of two homozygous T1 Csralf4 lines ( a ) and two homozygous T1 Csralf19 lines ( d ). Target sequences and PAMs are indicated below the black and red lines, respectively. Deletions/insertions are indicated as red dashes/nucleotides, and deletion/insertion sizes (nucleotides) are marked after the sequence as a minus or plus, respectively. The right dotted box shows the corresponding protein premature termination. The blue/orange boxes indicate CsRALF4/CsRALF19 protein coding region, respectively, and the gray indicates missense sequences resulting from frameshift mutations. aa amino acid. b , e Mature fruits, corresponding longisection, and harvested seeds from reciprocal crosses between Csralf4 mutants ( b )/ Csralf19 mutants ( e ) and WT. Scale bars = 5 cm. c , f Quantitative analysis of seed number from ( b , e ). Upmost/lowest lines indicate the maximum/minimum values, box limits indicate the upper and lower quartiles, and lines in boxes indicate the median values of these data. From left to right, n = 6, 5, 4, 7, 5, 5, 7 mature fruits in ( c ) and 7, 5, 5, 7, 6, 6, 6 mature fruits in ( f ), respectively. * p < 0.05, ** p < 0.01 (two-sided Student’s t -test). Full size image Fig. 5: Reduced female fertility in Csralf4 Csralf19 double mutants. a Mutation forms of two homozygous T1 transgenic Csralf4 Csralf19 lines. The target sequence and PAM are indicated below a black and a red line, respectively. Deletions/insertions are indicated as red dashes/nucleotides, and deletion/insertion sizes (nucleotides) are marked after sequencing as a minus or plus, respectively. The right dotted box shows the corresponding protein premature termination. The blue/orange boxes indicate CsRALF4/CsRALF19 protein coding region, respectively, and the gray indicates missense sequences resulting from frameshift mutations. aa, amino acid. b Mature fruits and corresponding longisection from reciprocal crosses between Csralf4 Csralf19 mutants and WT. The corresponding seed numbers were shown at the bottom. Scale bars =  5 cm. c All plump seeds and fruit transections from WT self-crossing and Csralf4 Csralf19 hybridizing with WT pollens. Scale bars = 2 cm. d , e Quantitative analysis of seed number. From left to right, n = 7, 6, 7 mature fruits in ( d ) and 8, 5, 6 mature fruits in ( e ), respectively. f Aniline blue staining showing the ovule targeting in WT and Csralf4 Csralf19 mutant ovaries at 32 h after pollination with WT pollens by transverse (left) and longitudinal sections (right). Yellow stars indicate ovules targeted by pollen tubes. Scale bars = 500 μm. g Quantitative analysis of pollen tubes entering ovules in ( f ). n = 5, 5, 4 biologically independent samples. h Pollen tubes distribution at lateral- and terminal-TT (pointed by green boxes and blue boxes, respectively) in ovary transections from ( f ). Scale bars = 500 μm. I , j Quantitative analysis of pollen tube fluorescence intensity at lateral- ( i ) and terminal-TT ( j ) in ( h ). The fluorescence threshold is 20–255. n = 39, 32, 36 lateral TTs in ( i ), and 235, 141, 120 terminal TTs in ( j ), respectively. For these Box-plots, upmost/lowest lines indicate the maximum/minimum values, box limits indicate the upper and lower quartiles, and lines in boxes indicate the median values of these data. *** p < 0.001 (two-sided Student’s t -test). Full size image Besides, defects in male gametophytes were detected in Csralf4, Csralf19 single mutants, and Csralf4 Csralf19 double mutants. Pollen viability was significantly reduced in all mutants ( Csralf4 : 92.3 ± 2.2%, 92.9 ± 1.1%; Csralf19 : 92.7 ± 1.9%, 93.0 ± 1.4%; Csralf4 Csralf19 : 83.2 ± 4.3%, 81.8 ± 4.7%; all p < 0.001) as compared to WT (96.6 ± 0.8%) (Fig. 6a, b ). WT pollen tubes ruptured after reaching 242.9 ± 89.3 μm length, while pollens tubes in two Csralf4 lines ruptured precociously at length of 172.0 ± 71.6 μm and 183.6 ± 67.1 μm ( p < 0.001, Fig. 6a, c ). Similarly, Csralf19 pollen tube length was 115.2 ± 67.2 μm (#1) and 122.0 ± 77.3 μm (#2) versus WT 233.0 ± 80.2 μm ( p < 0.001, Fig. 6a, d ). In addition, the weakened fluorescence intensity by Aniline blue staining indicated poor extension of Csralf4 and Csralf19 pollen tubes in WT ovaries, especially at lateral- and terminal-TT (Fig. 6e ). In Csralf4 Csralf19 double mutants, pollen tubes burst immediately upon germination in vitro and on the stigmatic surface, which resembles the Arabidopsis ralf4 ralf19 mutant phenotypes (Fig. 6a, e ), suggesting the conserved function of CsRALF4/19 in pollen tube integrity [32] . Fig. 6: Abolished male fertility in Csralf4 Csralf19 double mutants. a Alexander staining of pollens (top row) and in vitro pollen germination assay (bottom row) of Csralf4 , Csralf19 and Csralf4 Csralf19 mutants. Scale bars = 100 μm. b–d Quantitative analysis of pollen viability ( b ) and pollen tubes length ( c , d ) from ( a ). n = 9, 3, 3, 3, 3, 3, 3 biologically independent samples in ( b ). Error bars represent mean ± SD. n = 115, 71, 48 pollen tubes in ( c ) and 240, 97, 83 pollen tubes in ( d ), respectively. *** p < 0.001 (two-sided Student’s t test). For these Box-plots, upmost/lowest lines indicate the maximum/minimum values, box limits indicate the upper and lower quartiles, and lines in boxes indicate the median values of these data. e Aniline blue staining showing the extension of pollen tubes by longitudinal (up) and transverse sections (bottom) in Csralf4 , Csralf19, and Csralf4 Csralf19 mutants. Composite images were integrated and spliced from local images taken separately. Scale bars = 500 μm. Full size image CsALC was selected during cucumber domestication Our findings showed the important function of CsALC in cucumber seed production and sustainable propagation. During cucumber domestication, the fruit is elongated while seed number per unit fruit length is generally decreased [33] . To explore any selection footprint on CsALC , the genomic region of CsALC plus its 3 kb promoter sequences (Chr02: 16738402–16744826) was analyzed in the published 115 cucumber accessions consisting of five populations: Indian wild genotypes (INW), Indian domestic (IND), Xishuangbanna (XSBN), East Asian (EA) and Eurasian (EU) [28] . The results showed that CsALC exhibited sharply reduced nucleotide diversity (π) in modern varieties (EA and EU), as compared to wild (INW) or semi-wild cucumber (XSBN) (Supplementary Fig. 8a ). We also calculated the pairwise difference in allele frequency (FST) between domesticated groups and wild population INW, the results showed that CsALC was selected in Xishuangbanna, East Asian and Eurasian groups (Supplementary Fig. 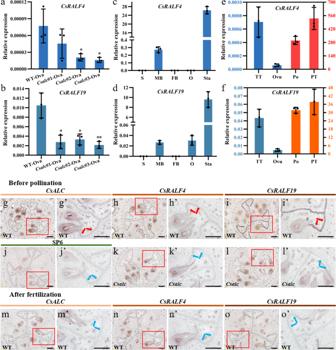Fig. 3: Reduced transcript accumulation ofCsRALF4andCsRALF19inCsalcovaries. a,bExpression ofCsRALF4(a) andCsRALF19(b) in unpollinated ovaries at anthesis of WT andCsalcmutants by qPCR. *p< 0.05, **p< 0.01 (two-sided Student’st-test).c,dCsRALF4(c) andCsRALF19(d) expression in different cucumber organs. S stems, MB male flower buds at stage 1050; FB female flower buds at stage 1050; O ovaries at anthesis; Sta stamens at anthesis.e,fCsRALF4(e) andCsRALF19(f) expression in female sporophytes and male gametophytes. TT ovary transmitting tract at anthesis, Ovu ovules at anthesis, Po pollens at anthesis, PT pollen tubes at 3 h after germination. The left/right vertical axis refers to the data of the blue/orange column, respectively, due to the magnitude difference of expression in different tissues.n= 3 biologically independent samples (a–f). The values were normalized with theCsUBI(CsaV3_5G031430) expression (a-f). Error bars represent mean ± SD (a–f).g–o’Transcript accumulation ofCsALC(g,g’,m,m’),CsRALF4(h,h’,k,k’,n,n’), andCsRALF19(i,i’,l,l’,o,o’) at transmitting tract of unpollinated WT andCsalcovaries (g–l’) and fertilized WT ovaries one day after anthesis (32 h after pollination) (m–o’) by in situ hybridization.j–j’SP6, SenseCsALCprobe was hybridized as the negative control.g’–o’are enlargements of red boxes in (g–o). Red arrows indicate transcript signals at lateral- and terminal-TTs in WT before pollination, and blue arrows refer to the weakened transcript signals at lateral- and terminal-TTs inCsalcmutants, or in WT after fertilization. Scale bars = 500 μm. The experiment was repeated three times with similar results. 8b ), implying the importance of CsALC in cucumber domestication and breeding. The ovary encloses and nourishes ovules, and ample evidence suggested that the ovary must provide an environment that supports pollen tube growth and guidance to the ovule [34] . Some female molecules, e.g. Ca 2+ ions [35] , γ aminobutyric acid (GABA) [36] , [37] , brassinosteroids [38] , carbohydrates [4] , and various peptides [39] , have been characterized to stimulate pollen germination and pollen tube growth in preovular guidance process. These early stages are generally regulated by sporophytic genes such as those in the transmitting tract, e.g., Transmitting-Tissue-Specific Arabinogalactan gene ( TTS ) in tobacco [40] , SPT [29] , HECATEs ( HEC1/2/3 ) [41] , HALF FILLED ( HAF ) [42] in Arabidopsis and CsSPT in cucumber [30] . In Csspt mutants, the dramatically decreased polysaccharide at the style transmitting tract led to much less pollen tubes penetrating into ovaries and thus reduced seed set and female fertility [30] . Unlike that stimulant molecules promote the movement of pollen tubes at stigma or styles at preovular guidance stage, the attractant cues secreted from ovules generally trigger the re-orientation of pollen tube during the ovular guidance process (late stage of pollen tube guidance), e.g. the roles of CRP peptide LUREs and synergid cells during short range attraction [6] , [20] , [43] . Meanwhile, male factors such as receptor PRK6 and ion transporters CHX21/23 mediate pollen tube responsive behavior and competence for ovular attractions [23] , [25] . However, none female sporophytic gene has been reported yet to positively regulate pollen tube re-orientation at the transition stage between preovular guidance and ovular guidance, namely the pollen tube emergence process. In this study, we identified a transmitting tract-expressed gene CsALC that participates in pollen tube emergence in cucumber. Loss-of-function Csalc mutants displayed almost absence of pollen tube distribution at terminal TT and thus nearly 95% reduction in female fertility (Fig. 1 ). The movement of pollen tubes from top to bottom within Csalc pistils appeared normal while extending pollen tubes within Csalc ovaries failed to turn towards ovules, showing a defect in pollen tube emergence from lateral-TT to terminal-TT (Figs. 2 and 7 ). Unlike the hollow pod in Arabidopsis , cucumber bears the fleshy fruit, in which the cell–cell communication of pollen–pistil interactions mainly occurs at the transmitting tracts. From the physiological and molecular evidence, we can speculate that the transmitting tract circumstance in Csalc mutants is altered, in which main component polysaccharides and two TT-expressed peptides CsRALF4 and CsRALF19 were reduced (Figs. 2 and 3 ). The changed TT circumstance may affect the diffusion or distribution of some unknown ovular attractant molecules at lateral and terminal TT in cucumber, causing unresponsive pollen tube behavior. Another possibility is that the absence of female-assisted molecules at TTs, like phytohormones, peptides, and glycoproteins, may blunt the pollen tube perception for ovular signals or affect the directional growth of pollen tubes. The successful guidance for pollen tubes not only requires the secreted attractants but also the competency control from female tissues for pollen tube behavior [34] . It was reported that an ovary-abundant chemical cue, methyl-glucuronosyl arabinogalactan (AMOR), can promote pollen tube competence to respond to ovular attractant LURE peptides in Torenia fournieri [34] . The third possibility is that the mutant TT in Csalc may modify pollen tube status to lose the directional growth capacity. It may be operated through pollen-specific unknown receptors, or those genes involved in localized vesicle traffic, actin dynamics, or ion balance (e. g. Arabidopsis CHX21 and CHX23 in K + homeostasis) that specify pollen tube tip growth and re-orientation [44] . Fig. 7: A working model for CsALC and CsRALF4/19 in pollen tube guidance in cucumber. In WT ovary, pollen tubes (in red) extend successively along the medial-, lateral- and terminal-TT and eventually enter ovules, producing hundreds of seeds per fruit in cucumber. In Csalc mutant, pollen tubes fail to re-orient to ovules and are blocked at the lateral TT, partially due to the decrease of CsRALF4/19 peptides, resulting in an approximately 95% reduction in seed number per fruit. In Csralf4 Csralf1 9 mutant, the reduced pollen tube extension and decreased ovule targeting efficiency leads to about a 60% reduction of seed number in fruit. The much fewer seeds in Csalc mutants than in Csralf4 Csralf1 9 mutants indicate there must be other downstream target genes. Full size image However, despite a similarly reduced extracellular matrix in Csspt ovaries, no pollen tube emergence defect was observed (Supplementary Fig. 9 ) [30] , suggesting the polysaccharides in TT may not be the critical factor required for proper pollen tube re-orientation. CsSPT mainly functions in the development of style TT that facilitates pollen tube extension from the stigma to the ovary. Mutation of CsSPT resulted in only upper portion ovules fertilized and thus a 60% reduction in seed set [30] . Considering Csspt Csalc double mutants displayed a complete loss of female fertility derived from the absence of TT, more severe than either Csspt or Csalc single mutants [30] , therefore, we conclude that CsALC and CsSPT have divergent functions in pollen tube guidance, while redundant roles in TT development in cucumber. Besides the extremely high enrichment in pollens, CsRALF4/19 were also expressed in female reproductive tissues in cucumber (Fig. 3 ). Knockout of both CsRALF4 and CsRALF19 resulted in pollen tube rupture prematurely and reduced female fertility from diminished pollen tube distribution at lateral and terminal-TT, and decreased ovule targeting efficiency (Fig. 5 ). These data suggested that in addition to the conserved function in pollen tube integrity by pollen-located CsRALF4/19 peptides [12] , [13] , the transmitting tract-expressed CsRALF4/19 peptides mediate pollen tube growth and extension in the cucumber ovary, probably by interaction with pollen tube-expressed RALF receptors similar to those in pollen tube integrity control [12] (Fig. 7 ). Expression analysis indicated the CRPs CsRALF4 / 19 transcripts were decreased in Csalc ovaries (Fig. 3 ). Although no direct interaction was found by yeast one hybrid, in vivo assay of N. benthamiana showed the positive regulation of CsALC on CsRALF4/19 expression, perhaps with the assistance of other cofactors (Supplementary Fig. 7 ). Interestingly, the expression of CsRALF4/19 was unchanged in the stamen of Csalc mutant (Supplementary Fig. 6 ), implying the positive regulations of CsRALF4/19 by CsALC is female specific. Considering the crossing data of male sterility and reduced female fertility in Csralf4 Csralf19 double mutants (Figs. 5 and 6 ), CsRALF4/19 may have distinct functions in male and female cells in cucumber. Notably, the phenotype of seed set decrease in Csralf4 Csralf19 double mutants was not as severe as that in Csalc mutants, indicating there are additional downstream genes of CsALC besides CsRALF4/19 during pollen tube guidance (Fig. 7 ). As the paralog of SPT, ALC originated from a gene duplication event prior to the emergence of the Brassicaceae [29] . In the dehiscent silique of Arabidopsis , ALC controls fruit opening by promoting cell differentiation at separation layers [27] . In the berry fruit of Solanaceae, transient knock-down of both ALC and SPT genes resulted in increased fruit lignification in tomato and pepper [45] . In the fleshy pepo fruit of Cucurbitaceae, our study showed the unique role of CsALC in female fertility via mediating pollen tube emergence in cucumber (Fig. 2 , Fig. 7 ). Therefore, ALC has undergone functional divergence in different fruit types. From an evolutionary point of view, however, ALC homologs from different species commonly contribute to sexual reproduction success, such as participating in fruit opening and thus facilitating seed dispersal in Arabidopsis [46] , or controlling pollen tube guidance and enabling seed genesis in cucumber. Interestingly, CsALC surrounding region is under-selected during the domestication process in cucumber (Supplementary Fig. 8 ). In wild cucumbers, seedy fruits are advantageous for species reproduction and survival. However, in cultivated cucumber, fruits with fewer seeds are preferred for easy consumption. Thus, the CsALC gene may be selected unconsciously during the long history of cucumber cultivation. Notably, a segment in the first exon of CsALC (not the bHLH domain) displayed no polymorphism among all the 115 cucumber germplasms examined, which encoded a serine that is highly conserved in the Cucurbitaceae family. The functions of this specific serine, as well as the key domestication regions of CsALC await further studies. Plant materials and growth conditions Cucumber ( Cucumis sativus L.) inbred line XTMC (North China type) was used in this study. Seeds were soaked and germinated in the dark at 28 °C, then grown in the soil in a growth chamber under a 16 h/8 h and 28 °C/22 °C day/night regime until the roots fully developed and true leaves expanded. Seedlings were then transplanted to a standard greenhouse in the experimental field of China Agricultural University, Beijing. Water and fertilizer management, and pest control were performed according to standard protocols. Gene cloning and structural analysis An 1140-bp fragment containing the complete CsALC coding sequence (CDS) was amplified from male flower buds and open male flowers, and the 351-bp length CsRALF4 CDS and 339-bp length CsRALF19 CDS were obtained in the same way with gene-specific primers (Supplementary Data 1 ), based on sequence information in CuGenDB ( http://cucurbitgenomics.org/ ). 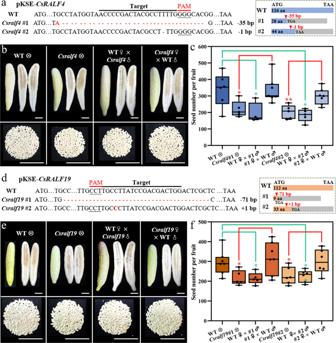Fig. 4: Decreased seed set inCsralf4andCsralf19single mutants. a,dMutation forms of two homozygous T1Csralf4lines (a) and two homozygous T1Csralf19lines (d). Target sequences and PAMs are indicated below the black and red lines, respectively. Deletions/insertions are indicated as red dashes/nucleotides, and deletion/insertion sizes (nucleotides) are marked after the sequence as a minus or plus, respectively. The right dotted box shows the corresponding protein premature termination. The blue/orange boxes indicate CsRALF4/CsRALF19 protein coding region, respectively, and the gray indicates missense sequences resulting from frameshift mutations. aa amino acid.b,eMature fruits, corresponding longisection, and harvested seeds from reciprocal crosses betweenCsralf4mutants (b)/Csralf19mutants (e) and WT. Scale bars = 5 cm.c,fQuantitative analysis of seed number from (b,e). Upmost/lowest lines indicate the maximum/minimum values, box limits indicate the upper and lower quartiles, and lines in boxes indicate the median values of these data. From left to right,n= 6, 5, 4, 7, 5, 5, 7 mature fruits in (c) and 7, 5, 5, 7, 6, 6, 6 mature fruits in (f), respectively. *p< 0.05, **p< 0.01 (two-sided Student’st-test). The gene structure was analyzed using the online software GSDS 2.0 ( http://gsds.gao-lab.org/ ). Phylogenetic trees construction To retrieve protein and CDS sequences for phylogenetic analysis, Arabidopsis SPT and ALC were used as queries to search against the genome database Phytozome ( https://phytozome.jgi.doe.gov/pz/portal.html ) and National Center for Biotechnology Information ( https://blast.ncbi.nlm.nih.gov/Blast.cgi ), using BLAST with a parameter of 1 × 10 −10 . Full-length protein sequences of sampled species were aligned using the program Muscle 3.6 ( http://www.drive5.com/muscle/ ), and the resulting alignment was manually adjusted in GeneDoc 3.2. Based on the protein alignment, a DNA matrix was produced by PAL2NAL ( http://www.bork.embl.de/pal2nal/ ). Protein sequences of RALFs from Arabidopsis and cucumber were obtained using the protein BLAST search in NCBI, TAIR ( https://www.Arabidopsis.org/ ), and CuGenDB. A phylogenetic tree was generated using the Neighbor-joining method and the bootstrap analysis with 1000 replicates in the MEGA-X. Multiple sequence alignment was performed using CLUSTALW in MEGA-X. Accession numbers of all sequences used for phylogenetic analysis are listed in Supplementary Data 2 . Subcellular localization of CsALC The full-length CDS of CsALC without termination codon was fused into the pUC-SPYNE vector to generate a CsALC-GFP in-frame fusion protein. The empty pUC-SPYNE vector was used as a positive control. Constructs were bombarded into onion epidermal cells using a PDS-1000/He particle delivery system (Bio-Rad) as described previously [47] . After incubation in the dark at 22 °C for 24 h, fluorescence signals were captured using a confocal laser-scanning microscope (Leica SP8, Germany) with 488 nm excitation wavelength. Quantitative real-time PCR The young leaves, stems, tendrils, male flower buds at stage 10, female flower buds at stage 10, male flowers, female flowers, ovaries and pollens, pollen tubes at 3 h after germination, transmitting tract, ovules were frozen in the liquid nitrogen and stored at −80 °C until use. Unless otherwise indicated, these reproductive tissues and organs were collected at anthesis (the day for pollination). Transmitting tracts and ovules were isolated from the middle parts of the ovary. Pollens from four male flowers were eluted in RNA-extracted lysis buffer. Pollens were cultured in liquid pollen germination medium [15% (w/v) sucrose, 0.01% (w/v) boric acid, 1 mM Ca(NO 3 ) 2 , pH 6.5] for 3 h and after centrifugal collection, pollen tubes were re-suspended in RNA-extracted lysis buffer. Total RNA was extracted with Trizol reagent as described in the manufacturer’s instructions (Promega, China, http://promega.bioon.com.cn/ ), and cDNA was synthesized using FastQuant RT Kit (Tiangen, China, http://www.tiangen.com/ ). Quantitative real-time PCR (qPCR) was performed using TB Green™ Premix Ex Taq™ (Takara, Japan, http://www.takarabiomed.com.cn/ ) on the Applied Biosystems 7500 real-time PCR system and Bio-RAD CFX384 system. Cucumber Ubiquitin extension protein ( CsUBI CsaV3_5G031430) was used as the internal reference gene [48] . The relative expression was calculated according to the comparative cycle threshold (CT) method [49] . Three biological replicates and three technical replicates were performed for each gene. Primer information is listed in Supplementary Data 1 . In situ hybridization The 25-day-old shoot apex, male and female flower buds, and ovaries at anthesis without pollination and at 32 h after pollination of XTMC and Csalc mutants were fixed with 3.7% formalin–acetic acid–alcohol (FAA) fixative. Sampling and recognition of flower buds at different developmental stages were referred to in the previous study [50] . Sense and antisense probes were amplified with gene-specific primers containing SP6 and T7 RNA polymerase binding sites, respectively. Sample fixation, sectioning, and hybridization were performed as described previously [51] . Primer information is listed in Supplementary Data 1 . Cucumber transformation The CRISPR-Cas9 knockout vector pKSE402 with GFP fluorescence screening marker is provided by Prof. Huang Sanwen. The guide RNA (gRNA) is designed in the Cas-Designer website ( http://www.rgenome.net/cas-designer/ ). Single target primers (for mutation of CsALC , CsRALF4 ) and double target primers (For simultaneous mutation of CsRALF4 and CsRALF19 ) were designed and synthesized according to the published methods [52] . Single target gRNA generated by denaturing annealed, and double target gRNAs by PCR amplification using vector pCBC-DT1T2 as template were respectively incorporated into vector pKSE402. Agrobacterium tumefaciens EHA105 carrying the recombinant vector was shake-cultured to OD 600 0.6–0.8, then adjusted to OD 600 0.2–0.3. The cucumber cotyledon explant was infected by Agrobacterium suspensions with a syringe under negative pressure. After 3 days of co-culture in darkness, explants were transferred to the medium for bud differentiation and bacteriostasis. After 3–4 weeks, the regenerated shoots with GFP fluorescence were screened under a fluorescence stereomicroscope (Filter Cube: Excitation filters 460–500 nm, Dichroic mirror 505 nm, and Barrier filters 510 nm). The homozygous T1 mutant seedlings without vector (GFP-free) were selected from T0 transgenic lines for further phenotypic analysis and data statistics. Details about cucumber tissue culture refer to the previous study [53] . Alexander staining for pollen viability Stamens from open male flowers, at least 3 for each plant, were washed to make pollen suspension (each flower stamen with 200 μL H 2 O). 5 μL pollen suspension and 15 μL Alexander dye were mixed on the slide and stained for 2 min. The pollen grains stained with purplish red under the microscope indicate the viable pollens. Each biological replicate counted at least 5 fields. in vitro pollen germination Pollen grains from open male flowers were lightly swept into the pollen germination medium [15% (w/v) sucrose, 0.01% (w/v) boric acid, 1 mM Ca(NO 3 ) 2 , and 0.5% (w/v) agar, pH 6.5] using a soft brush [54] . After being cultured in light and humid at 28 °C for 3 h, the germinating pollen tubes were observed and captured under microscope. The pollen tube germination percentage and pollen tube length were counted and measured in CellSens standard and ImageJ software [55] . At least three male flowers were counted for each mutant line and five fields were counted for each Petri dish. Pollen tube length longer than pollen grain diameter is determined as normal germination. Aniline blue staining of pollen tubes One female flower was pollinated with two male flowers. Pollinated excised pistils (with superior ovaries) were placed in Petri dishes and wetly cultured in a growth chamber under a 16 h/8 h and 28 °C/22 °C day/night regime. After 32 h, the pistils were sliced lengthwise or crosswise (about 0.5–1 mm in thickness) and fixed in 75% ethanol and 25% acetic acid solution for 3–6 h. After softened in 8 M NaOH for 3–6 h, the sample slices were stained with Aniline blue solution [0.1% (w/v) Aniline Blue in 0.1 M K 3 PO 4 ] for at least 2 h. The pistil slice was placed on a slide and the pollen tube extension in vivo was observed and photographed under a fluorescence microscope with excitation wavelength of 330–385 nm [56] . The pollen tube density in pistils was indicated by fluorescence intensity and quantitated in ImageJ software [55] . 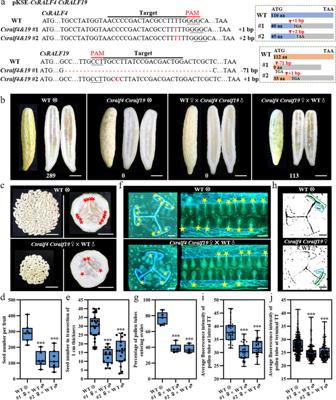Fig. 5: Reduced female fertility inCsralf4 Csralf19double mutants. aMutation forms of two homozygous T1 transgenicCsralf4 Csralf19lines. The target sequence and PAM are indicated below a black and a red line, respectively. Deletions/insertions are indicated as red dashes/nucleotides, and deletion/insertion sizes (nucleotides) are marked after sequencing as a minus or plus, respectively. The right dotted box shows the corresponding protein premature termination. The blue/orange boxes indicate CsRALF4/CsRALF19 protein coding region, respectively, and the gray indicates missense sequences resulting from frameshift mutations. aa, amino acid.bMature fruits and corresponding longisection from reciprocal crosses betweenCsralf4 Csralf19mutants and WT. The corresponding seed numbers were shown at the bottom. Scale bars =  5 cm.cAll plump seeds and fruit transections from WT self-crossing andCsralf4 Csralf19hybridizing with WT pollens. Scale bars = 2 cm.d,eQuantitative analysis of seed number. From left to right,n= 7, 6, 7 mature fruits in (d) and 8, 5, 6 mature fruits in (e), respectively.fAniline blue staining showing the ovule targeting in WT andCsralf4 Csralf19mutant ovaries at 32 h after pollination with WT pollens by transverse (left) and longitudinal sections (right). Yellow stars indicate ovules targeted by pollen tubes. Scale bars = 500 μm.gQuantitative analysis of pollen tubes entering ovules in (f).n= 5, 5, 4 biologically independent samples.hPollen tubes distribution at lateral- and terminal-TT (pointed by green boxes and blue boxes, respectively) in ovary transections from (f). Scale bars = 500 μm.I,jQuantitative analysis of pollen tube fluorescence intensity at lateral- (i) and terminal-TT (j) in (h). The fluorescence threshold is 20–255.n= 39, 32, 36 lateral TTs in (i), and 235, 141, 120 terminal TTs in (j), respectively. For these Box-plots, upmost/lowest lines indicate the maximum/minimum values, box limits indicate the upper and lower quartiles, and lines in boxes indicate the median values of these data. ***p< 0.001 (two-sided Student’st-test). 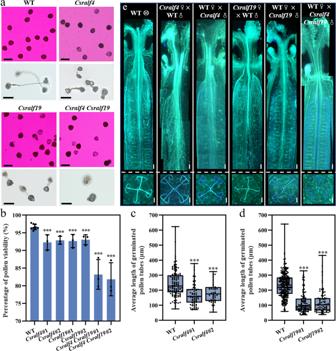Fig. 6: Abolished male fertility inCsralf4 Csralf19double mutants. aAlexander staining of pollens (top row) and in vitro pollen germination assay (bottom row) ofCsralf4,Csralf19andCsralf4 Csralf19mutants. Scale bars = 100 μm.b–dQuantitative analysis of pollen viability (b) and pollen tubes length (c,d) from (a).n= 9, 3, 3, 3, 3, 3, 3 biologically independent samples in (b). Error bars represent mean ± SD. n = 115, 71, 48 pollen tubes in (c) and 240, 97, 83 pollen tubes in (d), respectively. ***p< 0.001 (two-sided Student’sttest). For these Box-plots, upmost/lowest lines indicate the maximum/minimum values, box limits indicate the upper and lower quartiles, and lines in boxes indicate the median values of these data.eAniline blue staining showing the extension of pollen tubes by longitudinal (up) and transverse sections (bottom) inCsralf4,Csralf19,andCsralf4 Csralf19mutants. Composite images were integrated and spliced from local images taken separately. Scale bars = 500 μm. 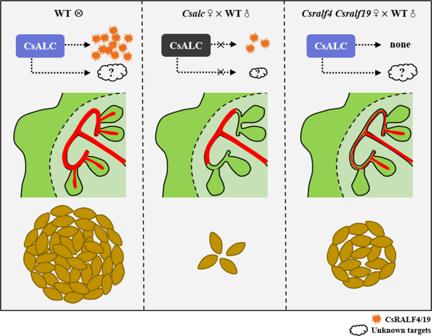Fig. 7: A working model for CsALC and CsRALF4/19 in pollen tube guidance in cucumber. In WT ovary, pollen tubes (in red) extend successively along the medial-, lateral- and terminal-TT and eventually enter ovules, producing hundreds of seeds per fruit in cucumber. InCsalcmutant, pollen tubes fail to re-orient to ovules and are blocked at the lateral TT, partially due to the decrease of CsRALF4/19 peptides, resulting in an approximately 95% reduction in seed number per fruit. InCsralf4 Csralf19 mutant, the reduced pollen tube extension and decreased ovule targeting efficiency leads to about a 60% reduction of seed number in fruit. The much fewer seeds inCsalcmutants than inCsralf4 Csralf19 mutants indicate there must be other downstream target genes. After fluorescence images were split into three channels, the red channel diagram was chosen and the fluorescence intensity was converted to the gray value, adjusted, and calculated in ImageJ software. Alcian blue staining of transmitting tracts Pistils at anthesis were fixed in 3.7% formaldehyde, 5% acetic acid, and 50% ethanol and subsequently dehydrated through ethanol series (50%, 70%, 85%, 95%, 100%, each 60 min), then hyalinized with xylene (50% 60 min, 100% 60 min three times) and embedded in paraffin. Samples (styles and ovaries) in paraffin were made for 10 μm thickness sections by microtome. After deparaffinization through xylene (10 min twice) and ethanol series (100%, 95%, 85%, 70%, 50%, each 5 min), sections were hydrated in water twice and stained with 0.5% Alcian blue solution (1 g Alcian blue 8GX in 200 mL H 2 O) for 30 min. After washing, sections were examined under microscopy [56] . The deeper blue refers to the higher acid polysaccharide content. Transcriptomic analysis Ovaries of WT and Csalc mutant at 32 h after pollination were collected for RNA-seq analysis. Three biological replicates were set. Illumina’s next-generation high-throughput sequencing platform and PE150 sequencing strategy were adopted. After quality control, clean read pairs were obtained and mapped to the cucumber genome sequence ( http://cucurbitgenomics.org/ Chinese long CDS V2). All genes were quantitatively analyzed to identify the differential genes. The cutoff for DEGs was at least a 2-fold change in expression and a false discovery rate (FDR) of <0.05 [57] (listed in Supplementary Data 3 ). Sequencing data were deposited with the Gene Expression Omnibus (GEO) database at the National Center for Biotechnology Information under accession number GSE182139. Yeast one-hybrid assay Vectors pB42AD and pLacZi2u were used for yeast one-hybrid assay. Plasmids for AD-fusions of CsALC were co-transformed with the LacZ reporters driven by two fragments from CsRALF4 or 3 fragments from CsRALF19 into the yeast strain EGY48. G-box elements were queried on CsRALF4/19 promoter and genomic region, as well as other 27 DEGs between Csalc mutant and WT in the PlantCARE website ( http://bioinformatics.psb.ugent.be/webtools/plantcare/html/ ). Yeast transformants were then selected on SD/-Trp-Ura agar plates for 4 days at 30 °C. The yeast transformants were further grown on SD/Gal/Raf/-Trp-Ura agar plates containing X-Gal (5-bromo-4-chloro-3-indolyl-β- d -galactopyranoside) for blue color development [58] . Yeast transformation was conducted as described in the Yeast Protocols Handbook (Clontech). LUC/REN assay for protein–DNA interactions in tobacco leaves The CsALC CDS was cloned into pGreenII 62-SK as effectors. The 1811 and 3326 bp sequences upstream of CsRALF4 and CsRALF19 coding regions were cloned into pGreenII 0800-LUC as reporters. The Agrobacterium GV3101 pSoup strain carrying the above recombinant vector (9: 1 effector: reporter construct cell culture mixture) was introduced into the half of a N. benthamiana leaf. The other half leaf was infiltrated with the strain carrying the empty effector and CsRALF4 / CsRALF19 reporter as a negative control. The activities of firefly luciferase (LUC) and Renilla reiformis luciferase (REN) were measured at 72 h after infiltration on a microplate reader instrument (Molecular Devices SpectraMax i3x, the USA). The ratio of LUC to REN was calculated as the measurement result of transcriptional activity of CsALC on CsRALF4 / 19 with eight biological replicates [59] . Nucleotide diversity and selective footprint analysis Published sequencing data of 115 cucumber germplasms with 37 East Asian (EA), 29 Eurasian (EU), 19 Xishuangbanna (XSBN), 13 Indian wild genotypes (INW), and 17 Indian domestic (IND) accessions were used in this analysis [28] . Nucleotide diversity was calculated as an π value for the five groups using VCFtools, which was further used to estimate the fixation index (FST) between EA/EU/XSBN/IND and the Indian wild counterparts (INW). Reporting summary Further information on research design is available in the Nature Portfolio Reporting Summary linked to this article.